Comprehensive interrogation of natural TALE DNA-binding modules and transcriptional repressor domains Transcription activator-like effectors are sequence-specific DNA-binding proteins that harbour modular, repetitive DNA-binding domains. Transcription activator-like effectors have enabled the creation of customizable designer transcriptional factors and sequence-specific nucleases for genome engineering. Here we report two improvements of the transcription activator-like effector toolbox for achieving efficient activation and repression of endogenous gene expression in mammalian cells. We show that the naturally occurring repeat-variable diresidue Asn-His (NH) has high biological activity and specificity for guanine, a highly prevalent base in mammalian genomes. We also report an effective transcription activator-like effector transcriptional repressor architecture for targeted inhibition of transcription in mammalian cells. These findings will improve the precision and effectiveness of genome engineering that can be achieved using transcription activator-like effectors. Transcription activator-like effectors (TALEs) are bacterial effector proteins found in Xanthamonas sp. and Ralstonia sp . Each TALE contains a DNA-binding domain consisting of 34 amino-acid tandem repeat modules, where the twelfth and thirteenth residues of each module, referred to as repeat-variable diresidues (RVDs), specify the target DNA base [1] , [2] . Four of the most abundant RVDs from naturally occurring TALEs have established a simple code for DNA recognition (for example, NI for adenine, HD for cytosine, NG for thymine, and NN for guanine or adenine) [1] , [2] . Using this simple code, TALEs have been developed into a versatile platform for achieving precise genomic and transcriptomic perturbations across a diverse range of biological systems [3] , [4] , [5] , [6] , [7] , [8] . However, two limitations remain: first, an RVD capable of robustly and specifically recognizing the DNA base guanine—a highly prevalent base in mammalian genomes [9] —is lacking; second, a viable TALE transcriptional repressor for mammalian applications has remained elusive, but would be highly desirable for a variety of synthetic-biology and disease-modelling applications [9] . To address these two limitations, we conducted a series of screens and found that of all naturally occurring TALE RVDs, the previously unidentified RVD Asn-His (NH) can be used to achieve guanine-specific recognition. Furthermore, we show that the mSin interaction domain (SID) [10] can be fused to TALEs to facilitate targeted transcriptional repression of endogenous mammalian gene expression. These advances further improve the power and precision of TALE-based genome engineering technologies, enabling efficient bimodal control of mammalian transcriptional processes. Screening of novel TALE RVDs Previously, the RVD NK was reported to have more specificity for guanine than NN [4] . However, recent studies have shown that substitution of NK with NN leads to substantially lower levels of activity [11] . To identify a more specific guanine-binding RVD with higher biological activity, we identified and evaluated a total of 23 naturally occurring RVDs ( Fig. 1 ) from the set of known Xanthomonas TALE sequences in Genbank. In order to directly compare the DNA-binding specificity and activity of all RVDs in an unbiased manner, we designed a set of 23 12.5-repeat TALEs where we systematically substituted RVDs 5 and 6 with the 23 naturally occurring RVDs (RVD-TALEs; Fig. 1a ). This design allowed us to maintain a consistent RVD context surrounding the two varied RVD positions. In addition, we fused a Gaussian luciferase gene ( Gluc ) with a 2A peptide linker to the RVD-TALEs to control for the differences in TALE protein expression levels ( Fig. 1a ). We used each RVD-TALE (for example, NI-TALE, HD-TALE, and so on) to assess the base preference and activity strength of its corresponding RVD—this is measured by comparing each RVD-TALE's ability to activate transcription from each of the four base-specific Cypridina luciferase reporter (Cluc) plasmids with A, G, T and C substituted in the sixth and seventh positions of the TALE-binding site (A-, G-, T- or C-reporters; Fig. 1a ). 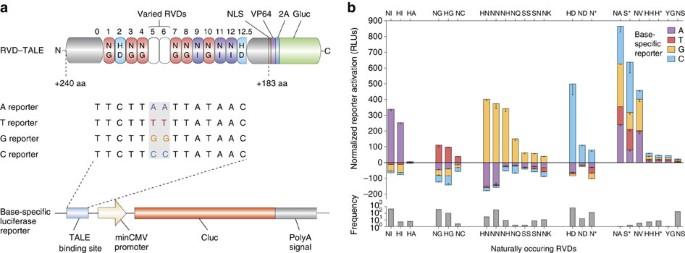Figure 1: Identification of an optimal guanine-specific RVD. (a) Design of the TALE RVD screening system. Each RVD-screening TALE (RVD-TALE) contains 12.5 repeats with RVDs 5 and 6 substituted with the 23 naturally occurring RVDs, and is fused to aGaussialuciferase gene via a 2A peptide linker. The truncations used for the TALE is marked at the amino and carboxy termini with numbers of amino acids (aa) retained (top). Four different base-specific reporters with A, T, G and C substituted in the sixth and seventh nucleotides of the binding site are used to determine the base specificity of each RVD (middle). Each reporter is constructed by placing the TALE-binding site upstream of a minimal CMV promoter drivingCypridinaluciferase (bottom). (b) Base preference of each natural RVD (top) is determined by measuring the levels of relative luminescence unit (RLU) for each base-specific reporter after background subtraction and normalization based on TALE protein expression level (top). We clustered RVDs according to their base preference after performing one-way ANOVA tests on each RVD. For RVDs with a single statistically significant reporter activity (P<0.05, one-way ANOVA), we plotted the reporter activity of the preferred base above thexaxis, whereas the reporter activities for the non-preferred bases are shown below thexaxis as negative. We clustered and ranked the RVDs without a single preferred base according to their total activity level. The abundance of each RVD in natural TALE sequences, as determined using all availableXanthomonasTALE sequences in GenBank, is plotted on a log scale (bottom). All bases in the TALE-binding site are color-coded (purple for A, red for T, orange for G and blue for C). NLS, nuclear localization signal; VP64, VP64 viral activation domain; 2A, 2A peptide linker; Gluc,Gaussialuciferase gene; minCMV, minimal CMV promoter; Cluc,Cypridinaluciferase gene; polyA signal, poly-adenylation signal. All results are collected from three independent experiments in HEK 293FT cells. Error bars indicate s.e.m.;n=3. Figure 1: Identification of an optimal guanine-specific RVD. ( a ) Design of the TALE RVD screening system. Each RVD-screening TALE (RVD-TALE) contains 12.5 repeats with RVDs 5 and 6 substituted with the 23 naturally occurring RVDs, and is fused to a Gaussia luciferase gene via a 2A peptide linker. The truncations used for the TALE is marked at the amino and carboxy termini with numbers of amino acids (aa) retained (top). Four different base-specific reporters with A, T, G and C substituted in the sixth and seventh nucleotides of the binding site are used to determine the base specificity of each RVD (middle). Each reporter is constructed by placing the TALE-binding site upstream of a minimal CMV promoter driving Cypridina luciferase (bottom). ( b ) Base preference of each natural RVD (top) is determined by measuring the levels of relative luminescence unit (RLU) for each base-specific reporter after background subtraction and normalization based on TALE protein expression level (top). We clustered RVDs according to their base preference after performing one-way ANOVA tests on each RVD. For RVDs with a single statistically significant reporter activity ( P <0.05, one-way ANOVA), we plotted the reporter activity of the preferred base above the x axis, whereas the reporter activities for the non-preferred bases are shown below the x axis as negative. We clustered and ranked the RVDs without a single preferred base according to their total activity level. The abundance of each RVD in natural TALE sequences, as determined using all available Xanthomonas TALE sequences in GenBank, is plotted on a log scale (bottom). All bases in the TALE-binding site are color-coded (purple for A, red for T, orange for G and blue for C). NLS, nuclear localization signal; VP64, VP64 viral activation domain; 2A, 2A peptide linker; Gluc, Gaussia luciferase gene; minCMV, minimal CMV promoter; Cluc, Cypridina luciferase gene; polyA signal, poly-adenylation signal. All results are collected from three independent experiments in HEK 293FT cells. Error bars indicate s.e.m. ; n =3. Full size image The 23 RVD-TALEs exhibited a wide range of DNA base preferences and biological activities in our reporter assay ( Fig. 1b ). In particular, NH- and HN-TALEs activated the guanine reporter preferentially and at similar levels as the NN-TALE. Interestingly, the NH-TALE also exhibited significantly higher specificity for the G-reporter than the NN-TALE (ratio of G- to A-reporter activations: 16.9 for NH-TALE and 2.7 for NN-TALE; Fig. 1b ), suggesting that NH might be a better RVD for targeting guanines. Our computational analysis of TALE-RVD specificity using a recently published crystal structure of TALE–DNA complex [12] also suggests that NH has a significantly higher affinity for guanine than NN ( Fig. 2 ). We found that substitution of NN with NH in one repeat within the TALE DNA-binding domain resulted in a gain of 0.86±0.67 kcal mol −1 in free energy (ΔΔ G ) in the DNA-bound state ( Fig. 2 ). 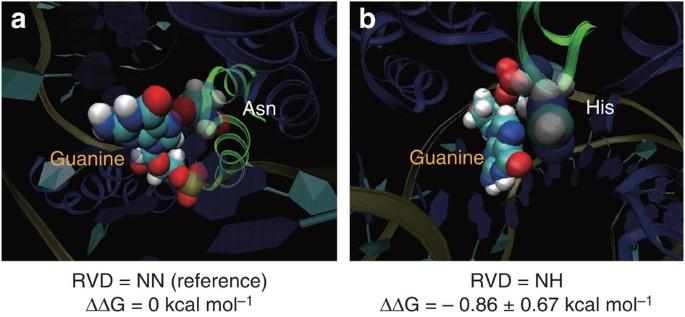Figure 2: Computational analysis of TALE RVD specificity. We performed extensive free FEP calculations for the relative binding affinities between the TALE and its bound DNA. Images show the three-dimensional configuration and results of the free-energy calculation for NN:G (a) and NH:G (b) interactions from one repeat in the TALE–DNA complex. The second amino acid (aa) of the guanine-recognizing RVD (that is, asparagine for RVD NN and histidine for RVD NH) and the guanine base of the bound double-stranded DNA are presented in space filling model and labelled. The free-energy calculation results are listed below their corresponding structures. Figure 2: Computational analysis of TALE RVD specificity. We performed extensive free FEP calculations for the relative binding affinities between the TALE and its bound DNA. Images show the three-dimensional configuration and results of the free-energy calculation for NN:G ( a ) and NH:G ( b ) interactions from one repeat in the TALE–DNA complex. The second amino acid (aa) of the guanine-recognizing RVD (that is, asparagine for RVD NN and histidine for RVD NH) and the guanine base of the bound double-stranded DNA are presented in space filling model and labelled. The free-energy calculation results are listed below their corresponding structures. Full size image Relative activity and specificity of guanine-binding RVDs To determine whether NH and HN are suitable replacements for NN as the G-specific RVD, we directly compared the specificity and activity strength of NN, NK, NH and HN. We chose two 18-base-pair (bp) targets within the CACNA1C locus in the human genome and constructed four TALEs for each target, using NN, NK, NH or HN as the G-targeting RVD ( Fig. 3a ). As the screening result ( Fig. 1b ) suggested that HN might be less discriminatory than NH when the targeted base is A instead of G, we first designed a luciferase assay to further characterize the G-specificity of each RVD. For each CACNA1C target site, we constructed four luciferase reporters: wild-type genomic target, and wild-type target with 2, 4 or all guanines mutated into adenines ( Fig. 3a , G-to-A reporters), and compared the activity of each TALE using these reporters ( Fig. 3a ). For both CACNA1C target sites, we found that the TALE with NH as the G-targeting RVD exhibited significantly higher specificity for guanine over adenine than the corresponding NK-, HN- and NN-containing TALEs. For target site 1, introduction of two G to A mutations led to 35.4% (TALE1-NN), 40.3% (TALE1-NK), 71.4% (TALE1-NH) and 30.8% (TALE1-HN) of reduction in luciferase activity. For target site 2, two G-to-A mutations led to 21.8% (TALE2-NN), 36.3% (TALE2-NK), 66.1% (TALE2-NH) and 13.9% (TALE2-HN) reduction in reporter activity. Additional G-to-A mutations resulted in further reduction of reporter activity, with NH exhibiting the highest level of discrimination ( Fig. 3a ). NH TALEs also exhibited significantly higher levels of reporter induction than NK TALEs (1.9 times for site 1 and 2.7 times for site 2), and comparable to NN and NH TALEs ( Fig. 3a ). Thus, we decided to focus on the RVDs NN, NK, NH and HN in subsequent experiments to assess their usefulness in modulating transcription at endogenous human genome targets. 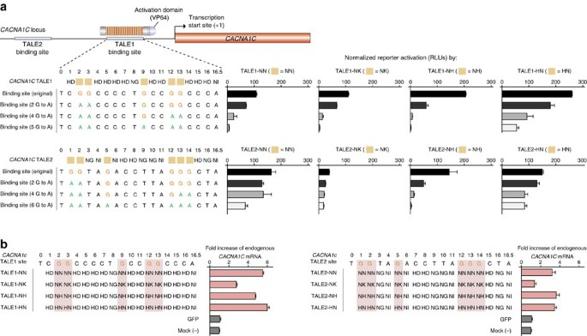Figure 3: Characterization of guanine-specific RVDs. (a) Specificity and activity of different guanine-targeting RVDs. Schematic showing the selection of two TALE-binding sites within theCACNA1Clocus of the human genome. The TALE RVDs are shown above the binding site sequences and yellow rectangles indicate positions of G-targeting RVDs (left). Four different TALEs using NN, NK, NH and HN as the putative G-targeting RVD were synthesized for each target site. The specificity for each putative G-targeting RVD is assessed using luciferase reporter assay, by measuring the levels of reporter activation of the wild-type TALE-binding site and mutant binding sites, with either 2, 4 or all guanines substituted by adenine. The mutated guanines and adenines are highlighted with orange and green, respectively. (b) Endogenous transcriptional modulation using TALEs containing putative G-specific RVDs. TALEs using NN, NK, NH and HN as the G-targeting RVD were synthesized to target two distinct 18-bp target sites in the humanCACNA1Clocus. Changes in messenger RNA (mRNA) are measured using qRT–PCR as described previously3. VP64, VP64 transcription activation domain. All results are collected from three independent experiments in HEK 293FT cells. Error bars indicate s.e.m.;n=3. Figure 3: Characterization of guanine-specific RVDs. ( a ) Specificity and activity of different guanine-targeting RVDs. Schematic showing the selection of two TALE-binding sites within the CACNA1C locus of the human genome. The TALE RVDs are shown above the binding site sequences and yellow rectangles indicate positions of G-targeting RVDs (left). Four different TALEs using NN, NK, NH and HN as the putative G-targeting RVD were synthesized for each target site. The specificity for each putative G-targeting RVD is assessed using luciferase reporter assay, by measuring the levels of reporter activation of the wild-type TALE-binding site and mutant binding sites, with either 2, 4 or all guanines substituted by adenine. The mutated guanines and adenines are highlighted with orange and green, respectively. ( b ) Endogenous transcriptional modulation using TALEs containing putative G-specific RVDs. TALEs using NN, NK, NH and HN as the G-targeting RVD were synthesized to target two distinct 18-bp target sites in the human CACNA1C locus. Changes in messenger RNA (mRNA) are measured using qRT–PCR as described previously [3] . VP64, VP64 transcription activation domain. All results are collected from three independent experiments in HEK 293FT cells. Error bars indicate s.e.m. ; n =3. Full size image Evaluation of guanine-binding RVDs at endogenous genome loci Using quantitative reverse transcriptase PCR, we further compared the performance of NN, NK, NH and HN for targeting endogenous genomic sequences. We tested the ability of NN, NK, NH and HN TALEs to activate CACNA1C transcription by targeting the two endogenous target sites ( Fig. 3b ). To control for differences in TALE expression levels, all TALEs were fused to 2A-GFP and exhibited similar levels of green fluorescent protein (GFP) fluorescence [3] . The endogenous activity of each TALE corresponded to the reporter assay. Both TALE1-NH and TALE2-NH were able to achieve similar levels of transcriptional activation as TALE1-NN and TALE2-NN (~5 fold and ~3 fold activation for targets 1 and 2, respectively) and twice more than TALE1-NK and TALE2-NK ( Fig. 3b ). Although TALE1-HN and TALE2-HN exhibited comparable activity with TALEs bearing RVDs NN and NH, the lack of specificity in distinguishing guanine and adenosine bases as shown in previous test ( Fig. 3a ) does not warrant the superiority of HN over existing guanine-binding RVDs. On the other hand, RVD NH exhibited similar levels of activity as NN and with higher specificity for guanine. Development of mammalian TALE transcriptional repressors Having identified NH as a more-specific G-recognizing RVD, we sought to develop a mammalian TALE-repressor architecture to enable researchers to suppress transcription of endogenous genes. TALE repressors have the potential to suppress the expression of genes as well as non-coding transcripts such as microRNAs, rendering it a highly desirable tool for testing the causal role of specific genetic elements. In order to identify a suitable repression domain for use with TALEs in mammalian cells, we used a TALE targeting the promoter of the human SOX2 gene to evaluate the transcriptional repression activity of a collection of candidate repression domains ( Fig. 4a ). We selected repression domains across a range of eukaryotic host species to increase the change of finding a potent synthetic repressor, including the PIE-1 repression domain (PIE-1) [13] from Caenorhabditis elegans , the QA domain within the Ubx gene (Ubx-QA) [14] from Drosophila melanogaster , the IAA28 repression domain (IAA28-RD) [15] from Arabidopsis thaliana , the SID [10] , Tbx3 repression domain (Tbx3-RD) and the Krüppel-associated box (KRAB) [16] repression domain from Homo sapiens ( Fig. 4b ). As different truncations of KRAB have been known to exhibit varying levels of transcriptional repression [16] , we tested three different truncations of KRAB ( Fig. 4c ). We expressed these candidate TALE repressors in HEK 293FT cells and found that TALEs carrying two widely used mammalian transcriptional repression domains, the SID [10] and KRAB [16] domains, were able to repress endogenous SOX2 expression, while the other domains had little effect on transcriptional activity ( Fig. 4c ). To control for potential perturbation of SOX2 transcription owing to TALE binding, expression of the SOX2-targeting TALE DNA-binding domain alone without any effector domain had no effect (similar to mock or expression of GFP) on the transcriptional activity of SOX2 ( Fig. 4c , null condition). As the SID domain was able to achieve 26% more transcriptional repression of the endogenous SOX2 locus than the KRAB domain ( Fig. 4c ), we decided to use the SID domain for our subsequent studies. 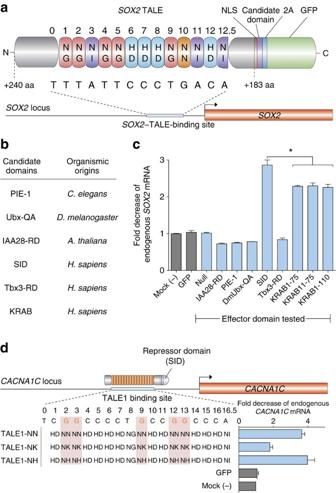Figure 4: Development of aTALE transcriptional repressor architecture. (a) Design ofSOX2TALE for TALE-repressor screening. A TALE targeting a 14-bp sequence within theSOX2locus of the human genome was synthesized as described previously3. (b) List of all repressors screened and their host origin (left). Eight different candidate repressor domains were fused to the C-term of theSOX2TALE. (c) The fold decrease of endogenous SOX2 messenger RNA (mRNA) is measured using qRT–PCR by dividing theSOX2mRNA levels in mock-transfected cells bySOX2mRNA levels in cells transfected with each candidate TALE repressor. (d) Transcriptional repression of endogenous CACNA1C. TALEs using NN, NK and NH as the G-targeting RVD were constructed to target a 18-bp target site within the humanCACNA1Clocus (site 1 inFig. 3). Each TALE is fused to the SID repression domain. NLS, nuclear localization signal; KRAB, Krüppel-associated box. All results are collected from three independent experiments in HEK 293FT cells. Error bars indicate s.e.m.;n=3. *P<0.05, Student'st-test. Figure 4: Development of aTALE transcriptional repressor architecture. ( a ) Design of SOX2 TALE for TALE-repressor screening. A TALE targeting a 14-bp sequence within the SOX2 locus of the human genome was synthesized as described previously [3] . ( b ) List of all repressors screened and their host origin (left). Eight different candidate repressor domains were fused to the C-term of the SOX2 TALE. ( c ) The fold decrease of endogenous SOX2 messenger RNA (mRNA) is measured using qRT–PCR by dividing the SOX2 mRNA levels in mock-transfected cells by SOX2 mRNA levels in cells transfected with each candidate TALE repressor. ( d ) Transcriptional repression of endogenous CACNA1C. TALEs using NN, NK and NH as the G-targeting RVD were constructed to target a 18-bp target site within the human CACNA1C locus (site 1 in Fig. 3 ). Each TALE is fused to the SID repression domain. NLS, nuclear localization signal; KRAB, Krüppel-associated box. All results are collected from three independent experiments in HEK 293FT cells. Error bars indicate s.e.m. ; n =3. * P <0.05, Student's t -test. Full size image To further test the effectiveness of the SID repressor domain for downregulating endogenous transcription, we combined SID with CACNA1C-target TALEs from the previous experiment ( Figs 3 and 4d ). Using quantitative reverse transcriptase PCR, we found that replacement of the VP64 domain on CACNA1C-targeting TALEs with SID was able to repress CACNA1C transcription. In addition, similar to the transcriptional activation study ( Fig. 3b , left), NH-containing TALE repressor was able to achieve a similar level of transcriptional repression as the NN-containing TALE (~4 fold repression), while the TALE repressor using NK was significantly less active (~2 fold repression, Fig. 4d ). These data demonstrate that SID is indeed a suitable repression domain, while also further supporting NH as a more suitable G-targeting RVD than NK. TALEs can be easily customized to recognize specific sequences on the endogenous genome, and can be used to target a diverse range of effector domains to specific genomic loci. Here, we conducted a series of screens to improve the specificity TALE-DNA recognition as well as expand the functionality of TALEs for modulating endogenous gene transcription. Our TALE RVD screening results identified a set of novel RVDs with useful activity and specificity. Among them, the RVD NH demonstrated increased specificity for recognizing guanine. While NK was previously shown to be able to target guanine specifically [17] , our endogenous gene modulation tests as well as a recent TALE nuclease study [11] have shown that TALEs employing NK to target guanine has less than half of the activity compared with TALEs using NN or NH. Our computational modelling result using the recently resolved crystal structure of a TALE–DNA complex [12] show that the imidazole ring on the histidine residue of the NH RVD has a more compact base-stacking interaction with the target guanine base ( Fig. 2 ), indicating that NH would be able to bind guanine more tightly than NN with a 0.86 ± 0.67 kcal/mol higher binding affinity and thus suggesting a possible mechanism for its increased specificity for guanine. Therefore based on all of these results from specificity and endogenous activity tests, the RVD NH seems to be a more suitable substitute for NN than NK when higher targeting specificity is desired. Further testing using additional endogenous genomic targets will help validate the broad utility of NH as a highly specific G-targeting RVD. In addition, the RVD NA exhibited similar levels of reporter activation for all four bases and may be a promising candidate for high efficiency targeting of degenerate DNA sequences in scenarios where non-specific binding is desired [18] . In addition, our screen of six different repressor domains across a range of host species resulted in the identification of two repressor domains capable of repressing mammalian transcription. The SID domain achieved the strongest level of repression at endogenous mammalian genomic loci. Having the ability to use TALEs to target transcriptional effectors may enable persistent epigenetic modification in the chromatin state of target loci in the endogenous genome. However, future studies will need to elucidate the mechanism of targeted transcriptional modulation by TALE transcription factors and their specificity. The identification of a more stringent G-specific RVD with uncompromised activity strength as well as a robust TALE-repressor architecture expands the utility of TALEs for probing mammalian transcription and genome function. Construction of TALE activators, repressors and reporters All TALE activators and repressors were constructed as previously described using a hierarchical ligation strategy [3] , [7] . Briefly, TALE monomers bearing different RVDs were amplified with a common set of primers to add unique ligation adapters [3] , [7] to enable ordered assembly of TALE DNA-binding repeats. Arrays of DNA-binding repeats were assembled according to the target TALE-binding sites and cloned into the destination vector [3] , [7] . The destination vector contains a strong mammalian promoter (EF1α or cytomegalovirus (CMV)) and the TALE backbone including the cloning sites for inserting customized arrays of TALE DNA-binding domains. The sequences for all constructs used in this study can be found in Supplementary Table S1 . To control for differences in the expression of each TALE, all TALEs are in-frame fused with the Gaussia luciferase ( Gluc ) gene via a 2A linker. The Gluc gene will be translated in an equimolar amount as TALEs. Truncation variants of the KRAB domain, the PIE-1 repression domain (PIE-1), the QA domain within the Ubx gene (Ubx-QA), the IAA28 repression domain (IAA28-RD), Tbx3 repression domain (Tbx3-RD) and the SID were codon optimized for mammalian expression and synthesized with flanking NheI and XbaI restriction sites (Genscript). All repressor domains were cloned into the TALE backbone by replacing the VP64 activation domain using Nhe I and Xba I restriction sites. To control for any effect on transcription resulting from TALE binding, we constructed expression vectors carrying the TALE DNA-binding domain alone using PCR cloning. The coding regions of all constructs were completely verified using Sanger sequencing. All luciferase reporter plasmids were designed and synthesized by inserting the TALE-binding site upstream of the minimal CMV promoter driving the expression of a Cypridina luciferase ( Cluc ) gene ( Fig. 1 ), similar to minCMV-mCherry reporter used in previous studies [3] . Cell culture and luciferase reporter activation assay Maintenance of human embryonic kidney cell line HEK 293FT (Invitrogen) were carried out with DMEM supplemented with 10% fetal bovine serum (HyClone), 2 mM GlutaMAX (Invitrogen), 100 U ml −1 penicillin and 100 μg ml −1 streptomycin, under 37 °C, 5% CO 2 incubation condition. Luciferase reporter assays were performed by co-transfecting HEK 293FT cells with TALE-2A-luciferase expression and luciferase reporter plasmids. In the case of the reporter-only control, cells were co-transfected with a control Gaussia luciferase plasmid (pCMV-Gluc, New England BioLabs). HEK 293FT cells were seeded into 24-well plates the day before transfection at densities of 2×10 5 cells per well. Approximately 24 h after initial seeding, cells were transfected using Lipofectamine2000 (Invitrogen) following the manufacturer's protocol. For each well of the 24-well plates 700 ng of dTALE and 50 ng of each reporter plasmids were used to transfect HEK 293FT cells. Dual luciferase reporter assays were carried out with the BioLux Gaussia luciferase flex assay kit and BioLux Cypridina luciferase assay kit (New England Biolabs) following the manufacturer's recommended protocol. Briefly, media from each well of transfected cells were collected 48 h after transfection. For each sample, 20 μl of the media were added into a 96-well assay plate and mixed with each one of the dual luciferase assay mixes. After brief incubation, as indicated in the manufacturer's protocol, luminescence levels of each sample were measured using the Varioskan flash multimode reader (Thermo Scientific). The activity of each TALE is determined by measuring the level of luciferase reporter induction and calculated as the level of Cluc induction in the presence of TALE activator minus the level of Cluc induction without TALE activator. The activity of each TALE is normalized to the level of TALE expression as determined by the Gluc activity level (each TALE is in-frame fused to 2A-Gluc), to control for differences in cell number, sample preparation, transfection efficiency and protein expression level. The concentration of all DNA used in transfection experiments were determined using gel analysis. We determined the base preference of each RVD according to the induction of each base-specific reporters by the corresponding RVD screening TALE (RVD-TALE, Fig. 1a ). Statistical analyses were performed using one-way analysis of variance (ANOVA) tests. Each RVD was tested by taking the reporter with the highest luciferase activity as the putative preferred base and comparing it with the remaining three bases as a group. For a given RVD, if the putative preferred base gave statistically significant test results ( P <0.05, one-way ANOVA), we classified that RVD as having a single preferred base, otherwise that RVD is tagged as not having a single preferred base. Endogenous gene transcriptional activation assay For the endogenous gene transcriptional level assay to test the biological activities of TALE activators and TALE repressors, HEK 293FT cells were seeded into 24-well plates. 800 ng of TALE plasmid was transfected using Lipofectamine2000 (Invitrogen) according to the manufacturer's protocol. Transfected cells were cultured at 37 °C for 72 h before RNA extraction. At least 100,000 cells were harvested and subsequently processed for total RNA extraction using the RNAeasyPlus Mini Kit (Qiagen). Complementary DNA was generated using the High Capacity RNA-to-cDNA Master Mix (Applied Biosystems) according to the manufacturer's recommended protocol. After cDNA synthesis, cDNA from each samples were added to the qRT–PCR assay with the Taqman Fast Advanced PCR Master Mix (Applied Biosystems) using a StepOne Plus qRT–PCR machine. The fold activation in the transcriptional levels of SOX2 and CACNA1C messenger RNA were detected using standard TaqMan Gene Expression Assays with probes having the best coverage (Applied Biosystems; SOX2 , Hs01053049_s1; CACNA1C , Hs00167681_m1). Computational analysis of RVD specificity To assess the guanine specificity of NH, we performed extensive computational simulations to compare the relative binding affinities between guanine and NN or NH using free-energy perturbation (FEP) [19] , [20] , a widely used approach for calculating binding affinities for a variety of biological interactions, such as ligand–receptor binding, protein–protein interaction and protein–nucleic acid binding [21] , [22] . We based our calculations on the recently released crystal structure of the TALE PthXo1 bound to DNA (PDB ID: 3UGM) [12] . We used a fragment of the crystal structure containing repeats 11–18 of PthXo1 (RVD sequence: HD[11]–NG[12]–NI[13]–HD[14]–NG[15]–NN[16]–NG[17]–NI[18], the position of each repeat is indicated by the number in square bracket) and the corresponding 18-bp double-stranded DNA molecule containing the TALE-binding sequence (5′-CTACTGTA-3′) in the centre to compare the binding affinities of RVDs NN, NK and NH for guanine. In order to have a 'smooth' transition from one residue to another, 20 perturbation windows with soft-core potentials have been used. For each mutation, at least five independent runs starting from different initial configurations are performed for better convergence for both the bound (TALE–DNA) and free (TALE-only) states in FEP, with 60+ ns molecular dynamics simulation time generated each for the underlying conformation space sampling (see ref. 23 for more details). The TALE–DNA complex is then solvated in a 66 Å×77 Å×51 Å water box, with 100 mM NaCl added to mimic the physiological environment. The total number of atoms in the simulation system is 26,700. The CHARMM22 force field and TIP3P water model were used for the simulation. As the 16th repeat in the structure is NN, we computationally mutated NN into NH or NK and calculated the binding affinity of each configuration (NN:G and NH:G). The affinity was calculated as the gain of free energy (ΔΔ G ) in the DNA-bound state taking NN:G as reference (ΔΔ G =0). How to cite this article: Cong, L. et al . Comprehensive interrogation of natural TALE DNA binding modules and transcriptional repressor domains. Nat. Commun. 3:968 doi: 10.1038/ncomms1962 (2012).